Double perovskites as a family of highly active catalysts for oxygen evolution in alkaline solution The electronic structure of transition metal oxides governs the catalysis of many central reactions for energy storage applications such as oxygen electrocatalysis. Here we exploit the versatility of the perovskite structure to search for oxide catalysts that are both active and stable. We report double perovskites (Ln 0.5 Ba 0.5 )CoO 3− δ (Ln=Pr, Sm, Gd and Ho) as a family of highly active catalysts for the oxygen evolution reaction upon water oxidation in alkaline solution. These double perovskites are stable unlike pseudocubic perovskites with comparable activities such as Ba 0.5 Sr 0.5 Co 0.8 Fe 0.2 O 3− δ which readily amorphize during the oxygen evolution reaction. The high activity and stability of these double perovskites can be explained by having the O p -band centre neither too close nor too far from the Fermi level, which is computed from ab initio studies. The discovery of new cost-effective and highly active catalysts for electrochemical energy conversion and storage is of prime importance to address climate change challenges and develop storage options for renewable energy production. Among the electrochemical processes, the oxygen evolution reaction (OER) on water oxidation is efficiency-limiting for direct solar [1] , [2] and electrolytic water splitting (H 2 O→H 2 +½ O 2 ) [3] , [4] , rechargeable metal-air batteries (M x O 2 →M x +O 2 ) and regenerative fuel cells [5] . Transition metal oxides such as ABO 3 perovskites composed of rare and alkaline earth (A) and 3d transition metal cations (B) are of particular interest as they have intrinsic activities comparable to the gold standards of OER catalysts such as IrO 2 and RuO 2 (ref. 4 ). Sabatier’s principle, which qualitatively describes that high catalytic activity can be obtained when adsorbed species bind to the surface neither too strongly nor too weakly, has been instrumental to fundamental understanding of OER mechanisms and the development of highly active catalysts. Unfortunately, the binding strength of oxygen molecules and reaction intermediate species [6] , [7] is difficult to assess experimentally. Instead, experimental studies have correlated with the intrinsic OER activities of transition metal oxides with parameters [8] , [9] , [10] that can be estimated and measured from experiments such as the e g orbital filling of transition metal ions [10] . The use of e g orbital filling as an OER activity descriptor identified an optimal e g orbital occupancy near unity and led to the identification of Ba 0.5 Sr 0.5 Co 0.8 Fe 0.2 O 3− δ (BSCF) with a record intrinsic OER activity [10] . However, BSCF particles readily become amorphous under OER conditions, producing Co-O motifs having local order with edge-sharing octahedra [11] , [12] similar to electrodeposited Co oxides such as Co-Pi [13] , [14] , [15] , during which the OER activity and electrochemical active surface area increase. Here we report that the intrinsic OER activities of (Ln 0.5 Ba 0.5 )CoO 3− δ are among the highest reported to date, with the most active (Pr 0.5 Ba 0.5 )CoO 3− δ in the series exhibiting activities greater than BSCF, the most active cubic perovskite. Unlike BSCF, these double perovskites are stable under OER conditions based on measurements from cyclic voltammetry (CV), galvanostatic testing and transmission electron microscopy (TEM) imaging. The physical origin of the high activity and stability of these Co-based double perovskites is compared with Co-based pseudocubic perovskites and discussed in term of e g filling of Co ions and the O p -band centre relative to the Fermi level as predicted from density functional theory (DFT). OER activity measurements In this study, we examine double perovskites with a formula unit of LnBaCo 2 O 5+ δ ′ (Ln=Pr, Sm, Gd and Ho and Ln), which can be written as (Ln 0.5 Ba 0.5 )CoO 3− δ ( δ ′=1−2 δ ) in the formula unit of pseudocubic perovskites. Because of the large difference in ionic radius between lanthanides and barium, double perovskites differ from cubic perovskites by the ordering of A-site cations along the c direction [16] , [17] . The difference in ionic radius and polarizability between lanthanides and barium tends to localize the oxygen vacancies in the lanthanide plane [16] , [18] , [19] ( Fig. 1a ), in contrast to the randomly distributed vacancies of pseudocubic perovskites [19] , [20] . The presence of oxygen vacancies induces a stabilization of the d xz and d yz and the d z 2 molecular orbitals in the t 2g and e g -parentage orbitals, respectively, which leads to the formation of an oxygen-deficient octahedral symmetry—the so-called square pyramidal symmetry ( C 4v ) in Fig. 1c . The concentration of oxygen vacancies and the cobalt oxidation state in double perovskites can be tuned by the nature of the lanthanide [16] and both are expected to influence the OER activity. 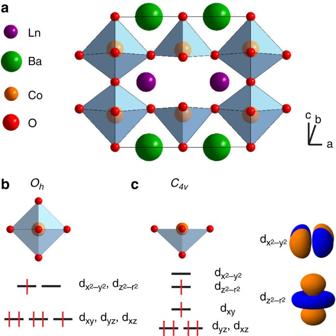Figure 1: Double perovskite crystal structure and cobalt crystal field. (a) Schematic representation of (Ln0.5Ba0.5)CoO3−δdouble perovskites (LnBaCo2O5+δ′withδ′=1−2δ) showing the ordering of Ln and Ba cations and the formation of oxygen deficiency in the LnO1−δplanes. This ordering is reflected by the doubling of thecparameter compared with ideal cubic perovskites, resulting inap×ap× 2aplattice parameters (apbeing the lattice parameter of cubic perovskite indexed in Pm-3m space group). The structure has (b) octahedral (Oh) and (c) square pyramidal (C4v) symmetry for Co ions, with different crystal-field splitting ofd-electron states for the different coordination symmetries. Figure 1: Double perovskite crystal structure and cobalt crystal field. ( a ) Schematic representation of (Ln 0.5 Ba 0.5 )CoO 3− δ double perovskites (LnBaCo 2 O 5+ δ ′ with δ ′=1−2 δ ) showing the ordering of Ln and Ba cations and the formation of oxygen deficiency in the LnO 1− δ planes. This ordering is reflected by the doubling of the c parameter compared with ideal cubic perovskites, resulting in ap × ap × 2 ap lattice parameters ( ap being the lattice parameter of cubic perovskite indexed in Pm-3m space group). The structure has ( b ) octahedral ( O h ) and ( c ) square pyramidal ( C 4v ) symmetry for Co ions, with different crystal-field splitting of d -electron states for the different coordination symmetries. Full size image (Ln 0.5 Ba 0.5 )CoO 3− δ (Ln=Pr, Sm, Gd and Ho) exhibited comparable OER activities from CV measurements, which were collected from oxide thin films supported on glassy carbon electrodes in O 2 -saturated 0.1 M KOH ( Fig. 2a ). (Pr 0.5 Ba 0.5 )CoO 3− δ was found to have the lowest voltage for the onset of oxidation current, indicative of the highest OER activity. The intrinsic OER activities normalized to the true oxide surface areas, which were estimated from Brunauer, Emmet and Teller (BET) measurements, are shown as a function of potential in Fig. 2b . Not only are the OER activities of these double perovskites one order of magnitude higher than that of LaCoO 3 (LCO), but they are also comparable to that of BSCF [10] , [11] and SrCo 0.8 Fe 0.2 O 3− δ (SCF) [11] , the most active OER catalysts known to date. In addition, Tafel slopes of the double perovskites (~60 mV per decade) are comparable to those of La 1− x Sr x CoO 3− δ (ref. 11 ) and Co-Pi [21] reported previously. Moreover, substituting cobalt with iron in the double perovskite structure, such as (Pr 0.5 Ba 0.5 )Co 1− x Fe x O 3− δ (with x =0.25 and 0.5) had negligible effect on the OER activity ( Supplementary Fig. S1 ). 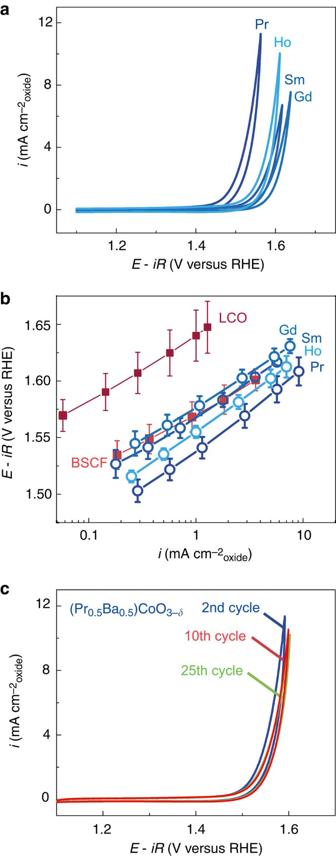Figure 2: Oxygen evolution activities of double perovskites. (a) Cyclic voltamograms of (Ln0.5Ba0.5)CoO3−δwith Ln=Pr, Sm, Gd and Ho (LnBaCO2O5+δ′withδ′=1−2δ), where measurements were performed using ink-casted oxides (containing Nafion and acetylene black carbon) with an oxide loading of 0.25 mg cm−2disksupported on a glassy carbon electrode in O2-saturated 0.1 M KOH electrolyte) with a scanning rate of 10 mV s−1. (b) Intrinsic OER activities normalized by the true oxide surface area, which were obtained from averaging currents in the forward and backward scans of the second cycle and subtracting the ohmic losses. The OER activities of Ba0.5Sr0.5Co0.8Fe0.2O3−δ(BSCF) and LaCoO3−δ(LCO) are included for comparison. Error bars represent s.d. from at least four independent measurements. (c) The 2nd, 10th and 25th CV scans of (Pr0.5Ba0.5)CoO3−δ. Figure 2: Oxygen evolution activities of double perovskites. ( a ) Cyclic voltamograms of (Ln 0.5 Ba 0.5 )CoO 3− δ with Ln=Pr, Sm, Gd and Ho (LnBaCO 2 O 5+ δ ′ with δ ′=1−2 δ ), where measurements were performed using ink-casted oxides (containing Nafion and acetylene black carbon) with an oxide loading of 0.25 mg cm −2 disk supported on a glassy carbon electrode in O 2 -saturated 0.1 M KOH electrolyte) with a scanning rate of 10 mV s −1 . ( b ) Intrinsic OER activities normalized by the true oxide surface area, which were obtained from averaging currents in the forward and backward scans of the second cycle and subtracting the ohmic losses. The OER activities of Ba 0.5 Sr 0.5 Co 0.8 Fe 0.2 O 3− δ (BSCF) and LaCoO 3− δ (LCO) are included for comparison. Error bars represent s.d. from at least four independent measurements. ( c ) The 2nd, 10th and 25th CV scans of (Pr 0.5 Ba 0.5 )CoO 3− δ . Full size image (Ln 0.5 Ba 0.5 )CoO 3− δ were found to be stable under OER potentials unlike BSCF [11] , [12] . No significant changes in the CV data or in the capacitive current were detected during repeated CV scans ( Fig. 2c ). This observation is in contrast to considerable changes in the CV scans of LiCoPO 4 (ref. 21 ), LiCoO 2 (ref. 21 ) and (B)SCF [11] , [12] , where the near-surface regions or the bulk of oxide particles become amorphous. The stability of the double perovskites during OER was further supported by galvanostatic measurements. The results obtained from (Pr 0.5 Ba 0.5 )CoO 3− δ are shown in Supplementary Fig. S2 as an example, where no significant changes occur in the voltage ( Supplementary Fig. S2a ) or in the CVs ( Supplementary Fig. S2b ) recorded before and after galvanostatic testing of 5 mA cm −2 oxide for 2 h. Further evidence of the double perovskite stability against OER came from TEM imaging. Although the surfaces of as-prepared double perovskites are perfectly crystalline ( Fig. 2a and Supplementary Fig. S3 ), exposing the oxides to tetrahydrofuran (THF) during the electrode preparation for OER measurements appeared to induce a small degree of amorphization, as shown in Fig. 3b and Supplementary Fig. S4 . No further change in the surfaces of double perovskites was observed after OER measurements, where TEM imaging showed that the surfaces of (Pr 0.5 Ba 0.5 )CoO 3− δ after 25 CV scans ( Fig. 3c and Supplementary Fig. S5a ) and 2 h held at 5 mA cm −2 oxide ( Fig. 3d and Supplementary Fig. S5b ) were comparable to those only exposed to THF ( Fig. 3b ). The stability of the double perovskite structure during OER measurements was further supported by the presence of cation-ordering reflections in the fast Fourier transforms (marked by * in Fig. 3c and Supplementary Fig. S5a ) and X-ray diffraction (XRD) pattern of cycled electrodes ( Supplementary Fig. S6 ), unique to the double perovskite structure with space group Pmmm and having a unit cell of ap × ap × 2 ap . This observation indicates that no leaching of praseodymium or barium occurs during oxygen evolution, unlike in BSCF [11] , and that these double perovskites are stable under the OER conditions used in this study. 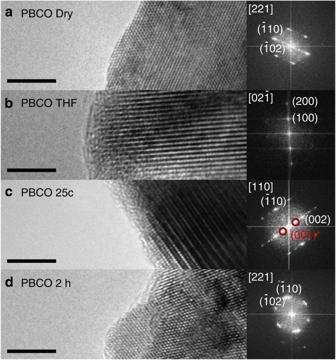Figure 3: Structure of double perovskites on oxygen evolution. High-resolution TEM images (scale bars, 5 nm) and fast Fourier transforms (FFTs) of (a) dry (Pr0.5Ba0.5)CoO3−δpowder, (b) (Pr0.5Ba0.5)CoO3−δexposed to tetrahydrofuran (THF), (c) (Pr0.5Ba0.5)CoO3−δcycled between 1.1 and 1.7 V versus reversible hydrogen electrode (RHE) at 10 mV s−1for 25 times and (d) (Pr0.5Ba0.5)CoO3−δgalvanostatically tested at 5 mA cm−2diskfor 2 h. (Pr0.5Ba0.5)CoO3−δmixed with Nafion and acetylene black carbon supported on a glassy carbon electrode with a loading of 0.25 mgoxidecm−2was tested in O2-saturated 0.1 M KOH electrolyte. FFTs images were indexed using Pmmm as space group andap×ap× 2aplattice parameters. Red circles indicate reflection that uniquely belongs to the double perovskite structure. Figure 3: Structure of double perovskites on oxygen evolution. High-resolution TEM images (scale bars, 5 nm) and fast Fourier transforms (FFTs) of ( a ) dry (Pr 0.5 Ba 0.5 )CoO 3− δ powder, ( b ) (Pr 0.5 Ba 0.5 )CoO 3− δ exposed to tetrahydrofuran (THF), ( c ) (Pr 0.5 Ba 0.5 )CoO 3− δ cycled between 1.1 and 1.7 V versus reversible hydrogen electrode (RHE) at 10 mV s −1 for 25 times and ( d ) (Pr 0.5 Ba 0.5 )CoO 3− δ galvanostatically tested at 5 mA cm −2 disk for 2 h. (Pr 0.5 Ba 0.5 )CoO 3− δ mixed with Nafion and acetylene black carbon supported on a glassy carbon electrode with a loading of 0.25 mg oxide cm −2 was tested in O 2 -saturated 0.1 M KOH electrolyte. FFTs images were indexed using Pmmm as space group and ap × ap × 2 ap lattice parameters. Red circles indicate reflection that uniquely belongs to the double perovskite structure. Full size image Correlation between OER activity and estimated e g filling To estimate the e g filling of cobalt ions in (Ln 0.5 Ba 0.5 )CoO 3− δ double perovskites, the cobalt oxidation and spin states are needed. The cobalt oxidation state was determined by iodometric and Mohr’s salt titrations, which was further confirmed by Co K-edge X-ray absorption spectroscopy (XAS, see Methods). The cobalt oxidation state was found to increase with increasing lanthanide ionic radius in Fig. 4a , which is in agreement with previous work by Maignan et al. [16] As Co K-edge XAS data showed comparable white line energies for Sm and Pr double perovskites, no significant change in the cobalt oxidation state was found for these two double perovskites ( Supplementary Figs S7a,S8 ). This is in contrast to the large difference obtained by chemical titration ( Fig. 4a ). The poor sensitivity of Co K-edge XAS for the oxidation state of cobalt greater than 3+ can be attributed to higher hybridization of Co-O bonds [22] (Estimating hybridization of transition-metal and oxygen states in perovskites from O K-edge X-ray absorption spectroscopy, manuscript in preparation) in the Pr double perovskite than the Sm double perovskite, which is supported by O K-edge XAS measurements discussed below. 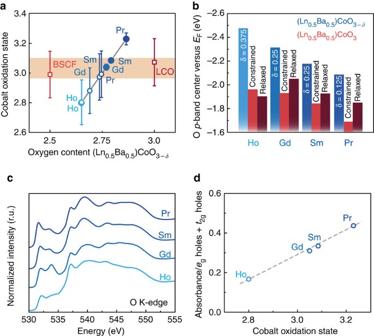Figure 4: Influence of lanthanides on electronic structure. (a) Cobalt oxidation obtained by chemical titration (closed symbols) and by XAS at the Co K-edge (open symbols) plotted versus the oxygen content for (Ln0.5Ba0.5)CoO3−δ(LnBaCo2O5+δ′withδ′=1−2δand Ln=Pr, Sm, Gd and Ho), Ba0.5Sr0.5Co0.8Fe0.2O3−δ(BSCF) and LaCoO3(LCO). The oxygen vacancy concentrationδwas directly calculated from the cobalt oxidation statexbyδ=(3.5−x)/2. The error bars in the oxidation state obtained by chemical titration represent the s.d. from at least three independent measurements. The errors in the oxidation state obtained by XAS were calculated by taking the root of the squared s.e. obtained by linear regression (see Methods). (b) The computed Op-band centre versus the Fermi level for the nonstoichiometric (Ln0.5Ba0.5)CoO3−δdouble perovskites (havingδconstrained to the values obtained from chemical titration) and stoichiometric (Ln0.5Ba0.5)CoO3in the constrained or relaxed structure (seeSupplementary Information). (c) O K-edge XAS data of (Ln0.5Ba0.5)CoO3−δmeasured in the total electron yield mode. (d) Integrated intensities of the O K-edge pre-edge region normalized to oxygen content per formula unit and the nominal number of empty cobalt 3dstates in bothegandt2gsymmetry. Figure 4: Influence of lanthanides on electronic structure. ( a ) Cobalt oxidation obtained by chemical titration (closed symbols) and by XAS at the Co K-edge (open symbols) plotted versus the oxygen content for (Ln 0.5 Ba 0.5 )CoO 3− δ (LnBaCo 2 O 5+ δ ′ with δ ′=1−2 δ and Ln=Pr, Sm, Gd and Ho), Ba 0.5 Sr 0.5 Co 0.8 Fe 0.2 O 3− δ (BSCF) and LaCoO 3 (LCO). The oxygen vacancy concentration δ was directly calculated from the cobalt oxidation state x by δ =(3.5− x )/2. The error bars in the oxidation state obtained by chemical titration represent the s.d. from at least three independent measurements. The errors in the oxidation state obtained by XAS were calculated by taking the root of the squared s.e. obtained by linear regression (see Methods). ( b ) The computed O p -band centre versus the Fermi level for the nonstoichiometric (Ln 0.5 Ba 0.5 )CoO 3− δ double perovskites (having δ constrained to the values obtained from chemical titration) and stoichiometric (Ln 0.5 Ba 0.5 )CoO 3 in the constrained or relaxed structure (see Supplementary Information ). ( c ) O K-edge XAS data of (Ln 0.5 Ba 0.5 )CoO 3− δ measured in the total electron yield mode. ( d ) Integrated intensities of the O K-edge pre-edge region normalized to oxygen content per formula unit and the nominal number of empty cobalt 3 d states in both e g and t 2g symmetry. Full size image Unfortunately, it is not straightforward to estimate the cobalt spin states in double perovskites because of the presence of O h and C 4v symmetries and multiple spin configurations [16] , [18] , [19] , [20] ( Fig. 1 ). Increasing the oxygen content from the Ho to Pr double perovskite leads to a greater number of Co 3+ in O h symmetry at the expense of C 4v symmetry, whereas the accompanied increase of the Co oxidation state reduces the number of Co 2+ and increases the number of Co 3+ and Co 4+ . By a first approximation, these double perovskites were selected to have the following spin states based on previous studies [20] , [23] , [24] : Co 2+ (3 d 7 ) having high spin in the C 4v symmetry because of polarizability and steric issues [25] ; Co 3+ (3 d 6 ) having intermediate spin in the O h and C 4v ; and Co 4+ (3 d 5 ) stabilized in high spin in the O h symmetry [26] ( Supplementary Fig. S9 ). Such assignments give rise to the e g occupancy of cobalt in these double perovskites near unity, having values from ~1.1 to ~1.3 ( Supplementary Fig. S9 ). The exceptionally high OER activities of these double perovskites, with their estimated e g values near unity ( Supplementary Fig. S10 ), support the design principle proposed by Suntivich et al. [10] , where the OER activity of perovskites peaks near e g occupancy of ~1.2. Correlation between OER activity and computed O p -band Despite its utility, the e g -filling estimation of cobalt ions is inferred from previous studies [10] , [27] and cannot be measured or computed directly. The presence of multiple spin states of cobalt ions in these double perovskites further introduces ambiguities in the estimation of e g filling. Recent studies [28] have shown that the computed O p -band centre relative to the Fermi level of perovskites scales linearly with the energy of oxygen vacancy formation and the oxygen surface exchange kinetics at elevated temperatures. We here report the O p -band centre relative to the Fermi level of perovskites as an alternative descriptor for the OER activities of perovskites in alkaline solution in an analogous role as the d -band centre for noble metal catalysts [29] , [30] . The O p -band centre was computed from DFT and details for the calculations can be found in the Supplementary Information . Owing to the strong correlation error present in standard DFT-generalized gradient approximation calculations of the transition metal 3 d -band, which was recently shown to be important for describing the OER activities of Co oxides [31] , the more delocalized nature of the O p -band more accurately captures the electronic structure characteristics of oxides critical to catalysis while still reflecting the metal d -character through hybridized density of states ( Fig. 5a ). 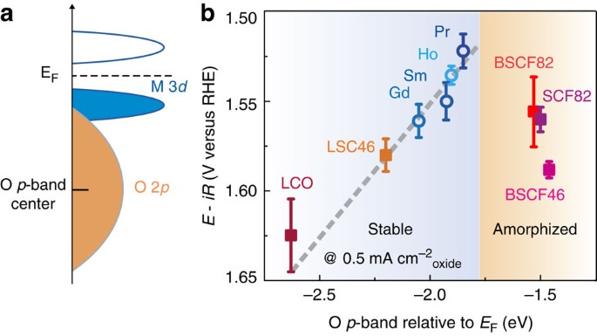Figure 5: Computed oxygenp-band centre for oxygen evolution. (a) Schematic representation of the Op-band for transition metal oxides and (b) evolution of theiR-corrected potential at 0.5 mA cm−2oxideversus the Op-band centre relative toEF(eV) of (Ln0.5Ba0.5)CoO3−δwith Ln=Pr, Sm, Gd and Ho, for LaCoO3(LCO)11, La0.4Sr0.6CoO3−δ(LSC46)11, Ba0.5Sr0.5Co0.8Fe0.2O3−δ(BSCF82)11, Ba0.5Sr0.5Co0.4Fe0.6O3−δ(BSCF46)11and SrCo0.8Fe0.2O3−δ(SCF82)11. The Op-band centre relative to the Fermi level was computed by DFT for the fully oxidized and relaxed structure using the method described in Methods section. Error bars represent s.d. from at least four independent measurements. Figure 5: Computed oxygen p -band centre for oxygen evolution. ( a ) Schematic representation of the O p -band for transition metal oxides and ( b ) evolution of the iR -corrected potential at 0.5 mA cm −2 oxide versus the O p -band centre relative to E F (eV) of (Ln 0.5 Ba 0.5 )CoO 3− δ with Ln=Pr, Sm, Gd and Ho, for LaCoO 3 (LCO) [11] , La 0.4 Sr 0.6 CoO 3− δ (LSC46) [11] , Ba 0.5 Sr 0.5 Co 0.8 Fe 0.2 O 3− δ (BSCF82) [11] , Ba 0.5 Sr 0.5 Co 0.4 Fe 0.6 O 3− δ (BSCF46) [11] and SrCo 0.8 Fe 0.2 O 3− δ (SCF82) [11] . The O p -band centre relative to the Fermi level was computed by DFT for the fully oxidized and relaxed structure using the method described in Methods section. Error bars represent s.d. from at least four independent measurements. Full size image The O p -band centre relative to the Fermi level of (Ln 0.5 Ba 0.5 )CoO 3− δ double perovskites using the cobalt oxidation state and oxygen nonstoichiometry determined from chemical titration ( Fig. 4a ) was found to linearly increase with increasing cobalt oxidation from Ho to Pr, as shown in Fig. 4b . This uplift of the O p -band centre with increasing cobalt oxidation would enhance Co-O hybridization, which is supported by O K-edge XAS measurements. The hybridization of Co-O bonds was found to increase from Ho to Pr double perovskite based on the O K-edge XAS measurements. The pre-edge feature can be attributed to unoccupied O 2 p states resulting from the mixing between O 2 p and metal 3 d states, and its intensity is linear with the number of holes in the O 2 p -band [22] . The intensity of the pre-edge region (two peaks near ~532–534 eV) increases with increasing ionic radius of the lanthanide ( Fig. 4c and Supplementary Fig. S7b ). The hybridization of Co-O bonds of these double perovskites can be assessed by the integrated intensities of the pre-edge region normalized to oxygen content per formula unit and the nominal number of empty cobalt 3 d states in both e g and t 2g symmetry. The hybridization was shown to increase and scale with increasing cobalt oxidation state associated with greater ionic radius of lanthanide ( Fig. 4d ). The trend can be attributed to decreasing charge transfer gap between oxygen 2 p and cobalt 3 d states associated with increasing cobalt oxidation state [32] . Assuming the surface of the catalyst to be fully oxidized in KOH under OER conditions, DFT studies of the O p -band centre were then performed on stoichiometric (Ln 0.5 Ba 0.5 )CoO 3 double perovskites ( Supplementary Fig. S11 ). Having oxygen stoichiometry in the double perovskite structure without structural relaxation gave rise to the same trend as that found for nonstoichiometric (Ln 0.5 Ba 0.5 )CoO 3− δ , but the O p -band centre was much uplifted because of increasing oxygen content ( Fig. 4b ). In contrast, the O p -band centre peaks on (Gd 0.5 Ba 0.5 )CoO 3 in the relaxed structure. The change in the O p -band centre trend versus (Ln 0.5 Ba 0.5 )CoO 3 series in the fully relaxed stoichiometric double perovskite structure was found to result from distortion and rotation of Co-O octahedra caused by A-site and B-site ionic radii mismatch ( Supplementary Fig. S11 ), which alters the Co-O bond length and metal 3 d –oxygen 2 p orbital hybridization [33] , leading to an upshift of the O p -band centre of (Ho 0.5 Ba 0.5 )CoO 3 relative to the Fermi level relative to the other double perovskites. The intrinsic OER activities of cobalt-based double perovskites and pseudocubic perovskites, which can vary by ~2 orders of magnitude ( Fig. 2b ), were found to correlate with the computed O p -band centre relative to the Fermi level of the fully oxidized and relaxed structure, as shown in Fig. 5b . It is appropriate to use the fully oxidized and relaxed structure in this analysis as the surface of these oxides is expected to be fully oxidized in KOH under OER conditions. Moving the O p -band centre closer to the Fermi level from LCO to (Pr 0.5 Ba 0.5 )CoO 3 greatly increases the intrinsic OER activity in the left branch. However, further lifting the O p -band centre in BSCF [11] , [28] , Ba 0.5 Sr 0.5 Co 0.4 Fe 0.6 O 3 (BSCF46) [11] and SCF [11] did not result in any increase in the OER activity but decreased the oxide stability. No changes were found for the oxides on the left branch in Fig. 5b during OER, whereas rapid amorphization in the near-surface regions accompanied with leaching of A-site ions, having local structures resembling that of Co-Pi, was observed for oxides on the right branch [11] , [12] . We show double perovskites (Ln 0.5 Ba 0.5 )CoO 3− δ (with Ln=Pr, Sm, Gd and Ho) as a new family of highly active catalysts for OER in alkaline electrolyte, with comparable activities and enhanced stability relative BSCF—the most active catalyst reported to date [10] , [11] . Although the high activities of these double perovskites with e g filling of cobalt ions near unity is in agreement with the design principle of OER catalysts reported recently [10] , considerable ambiguities exist in the estimation of e g filling associated with the presence of two crystal fields (octahedral O h and square pyramidal C 4v ), multiple Co oxidation states and multiple spin states of Co 3+ ions in these double perovskites. In this study, we show that the computed O p -band centre relative to the Fermi level and parameters derived from this can be used as descriptors to screen the OER activity and stability of oxides. Moving the computed O p -band centre closer to the Fermi level can increase OER activities, but having computed O p -band centre too close to the Fermi level decreases oxide stability during OER. This trend is similar to the correlation previously established for oxygen reduction on perovskites at elevated temperatures [28] . The pseudocubic perovskites and double perovskites with the O p -band centre very close to the Fermi level not only have the highest OER activities in alkaline solution but also exhibit the highest activities for surface oxygen exchange kinetics upon oxygen reduction at elevated temperatures [34] , which highlights the importance of the oxide electronic structure on oxygen electrocatalysis. Future spectroscopic experiments of these oxides are needed to verify the computed O p -band centre trend in this study, and seek activity and stability descriptors that can be measured experimentally. Our study highlights the importance of controlling a transition metal oxide having the O p -band close to the Fermi level as a promising strategy to create highly active oxide catalysts for OER to enable the development of efficient, rechargeable metal-air batteries, regenerative fuel cells and other rechargeable air-based energy storage devices. Synthesis and bulk characterization Double perovskite catalysts (Ln 0.5 Ba 0.5 )CoO 3− δ (with Ln=Pr, Sm, Gd and Ho) and (Pr,Ba)Co 1− x Fe x O 3− δ were synthesized using a conventional solid-state route. Stoichiometric amounts of Ln 2 O 3 , BaCO 3 and Co 3 O 4 and Fe 2 O 3 previously dehydrated were thoroughly grounded and fired in air at 1,000 °C for 12 h. Products were ground and annealed in air at 1,100 °C for (Ln 0.5 Ba 0.5 )CoO 3− δ catalysts and 1,200 °C for (Pr 0.5 Ba 0.5 )Co 1− x Fe x O 3− δ ( x =0.25 and 0.5) for 24 h with intermediate grindings. All catalysts reported in this study are single phase, as analysed by XRD ( Supplementary Fig. S14 ), with lattice parameters consistent with those reported previously [16] . XRD measurements were performed using a PANalytical X’Pert Pro powder diffractometer in the Bragg–Brentano geometry using a Copper K α radiation, where data were collected using the X’Celerator detector in the 8°–80° window in the 2 θ range. The specific surface area of each oxide sample was determined using BET analysis on a Quantachrome ChemBET Pulsar from a single-point BET analysis performed after 12 h outgassing at 150 °C, which is reported in Supplementary Table S1 . The oxygen vacancy δ was deduced by the determination of the cobalt oxidation state by chemical titration. For Ln=Pr, Gd and Sm, the samples were dissolved in an acidic medium (3 N HCl) with an excess of Mohr salt (Fe 2+ ). The Co 4+ concentration was deduced from the amount of remaining Fe 2+ ions determined by the back titration with a 0.1-N K 2 Cr 2 O 7 solution. For Ln=Ho, the Co 3+ amount was deduced by iodometric titration. The sample was dissolved in an acidic medium (3 N HCl) with 10 ml of a 10% mass KI aqueous solution. The iodine I 2 produced by the reduction of Co 3+ was then back titrated with a 0.02-N Na 2 S 2 O 3 . The titration was repeated three or four times for each oxide, from which an average oxidation state and the s.d. as the error bar were obtained. Electrochemical measurements of OER activities Electrodes were prepared by drop-casting ink containing oxide catalyst powder on a glassy carbon electrode, as described previously [35] . The glassy carbon electrode surface (0.196 cm 2 ) was loaded with 0.25 mg oxide cm −2 and a mass ratio of 5:1:1 of oxide catalyst to acetylene black carbon to Nafion. OER measurements were also performed on oxides electrodes drop casted on carbon cloth (ELAT LT1400W), where a loading of 0.2 mg oxide cm −2 and a mass ratio of 5:1:1 of oxide catalyst to acetylene black carbon to Nafion were used. The background oxidation current was estimated by measuring a carbon cloth loaded with 0.04 mg Nafion cm −2 . Cycled oxide electrodes on carbon cloth were examined by XRD to examine the oxide stability during OER. OER measurements were performed with a rotating disk-electrode set-up using a glass electrochemical cell with saturated calomel reference electrode and Pt counter electrode. A 0.1-M KOH (99.99% purity, Sigma-Aldrich) electrolyte was prepared with deionized water (>18 MΩ cm). Oxygen was bubbled to ensure O 2 /HO − equilibrium at 1.23 V versus reversible hydrogen electrode (RHE). The potential was controlled using a Biologic SP-300 potentiostat. A scan rate of 10 mV s −1 was used for all CV and rotation was set to 1,600 r.p.m. The saturated calomel reference electrode was calibrated in the same electrolyte by measuring hydrogen oxidation/evolution at a platinum electrode and defining the point of zero current as 0 V versus reversible hydrogen electrode (RHE). OER kinetic currents was obtained by taking the average between forward and backward scans to remove capacitive current contribution, which was then corrected for ohmic losses. Ohmic losses were corrected by subtracting the ohmic voltage drop from the measured potential, using an electrolyte resistance determined by high-frequency alternating current impedance, where iR -corrected potentials are denoted as E − iR ( i as the current and R as the electrolyte resistance). Error bars represent s.d. from at least four independent measurements. Near-surface structures by TEM imaging TEM imaging was conducted on a JEOL 2010F transmission electron microscope operated at 200 KeV, which is equipped with a field-emission electron gun and an ultrahigh resolution pole piece, resulting in a point-to-point resolution of 1.9 Å. Fourier analysis was performed using the Gatan Digital Micrograph software v2.01 (Gatan). As-prepared samples were prepared by gently grinding oxide powder dispersed in THF solvent, which was then sonicated for few minutes. The dispersion was then drop casted on a lacy carbon grid. Samples of cycled electrode were prepared by swabbing the glassy carbon surface, which was previously washed with ethanol to remove KOH remaining on the surface. X-ray absorption measurements O K-edge XAS were collected in the electron yield mode at the spherical grating monochromator beamline at the Canadian Light Source. The spectra were first normalized by I 0 being measured with a gold mesh before the specimen and then normalized by subtraction of a constant before the edge, and then division by a suitable constant after the edge. XAS at the Co K-edge was collected in fluorescence yield mode at the National Synchrotron Lightsource. The energy scale was calibrated by simultaneously measuring BSCF with known inflection points [12] . The Co oxidation states were calculated by relating the edge position obtained by the integral method [36] with the known oxidation states of single-phase Co 2+ O, Co 2+ (OH) 2 , Co 2.6+ 3 O 4 and LiCoO 2 using linear regression. The errors in the edge position are estimated and the errors in the oxidation state were calculated by taking the root of the squared s.e. obtained by linear regression. DFT studies DFT calculations with the Hubbard U ( U eff =3.3 eV) correction [28] , [37] for the Co 3 d electrons were performed with the Vienna Ab initio Simulation Package [38] , [39] using the projector-augmented plane-wave method [40] . Exchange-correlation was treated in the Perdew–Wang-91 generalized gradient approximation [41] . Fully relaxed stoichiometric bulk perovskite calculations were simulated with 2 × 2 × 2 perovskite supercells. The double perovskites were simulated based on the reported ordered structures within the 2 × 2 × 2 perovskite supercell [16] , [18] . An effective O p -band centre was determined by taking the centroid of the projected density of states of O 2p states relative to the Fermi level. More details of the calculations are provided in the Supplementary Information . How to cite this article: Grimaud, A. et al. Double perovskites as a family of highly active catalysts for oxygen evolution in alkaline solution. Nat. Commun. 4:2439 doi: 10.1038/ncomms3439 (2013).